Myc inhibition is effective against glioma and reveals a role for Myc in proficient mitosis Gliomas are the most common primary tumours affecting the adult central nervous system and respond poorly to standard therapy. Myc is causally implicated in most human tumours and the majority of glioblastomas have elevated Myc levels. Using the Myc dominant negative Omomyc, we previously showed that Myc inhibition is a promising strategy for cancer therapy. Here, we preclinically validate Myc inhibition as a therapeutic strategy in mouse and human glioma, using a mouse model of spontaneous multifocal invasive astrocytoma and its derived neuroprogenitors, human glioblastoma cell lines, and patient-derived tumours both in vitro and in orthotopic xenografts. Across all these experimental models we find that Myc inhibition reduces proliferation, increases apoptosis and remarkably, elicits the formation of multinucleated cells that then arrest or die by mitotic catastrophe, revealing a new role for Myc in the proficient division of glioma cells. Gliomas are the most frequent primary tumours affecting the adult human central nervous system. The World Health Organization defines four brain tumour classes (I, II, III, IV) on the basis of their morphological features and predicted clinical behaviour. The most lethal is grade IV glioblastoma (GBM), with a median survival of only 15 months [1] , [2] . However, all grades respond poorly to conventional therapy [3] . Gliomas are presumed to arise from mature glia or neural stem cells and diffusely infiltrate the surrounding tissue [3] , making surgical resection very difficult. Gliomas may be astrocytic, oligodendritic or of mixed lineage and are all characterized by refractoriness to apoptosis and marked genomic instability, both of which are thought to contribute to their poor response to chemo- and radiotherapy [3] . Recurring alterations observed in gliomas include amplification and activating mutations of EGFR, precocious receptor tyrosine kinase signalling, deletion of NF1 and elevated levels of p21 ras signalling (reviewed in ref. 3 ). In particular, signalling through the Ras network is essential for both proliferation [4] and angiogenesis [5] of human malignant astrocytomas. Myc is a bHLHZip transcription factor, causally implicated in most human cancers [6] . Myc controls diverse cellular functions, including cell growth and proliferation, differentiation and programmed cell death. Its expression in normal cells is tightly regulated by mitogen availability but this control is compromised in tumour cells, either as a consequence of constitutive upstream oncogenic signals or direct mutation in the myc genes themselves [7] . Myc expression correlate with glioma grade [8] and some 60–80% of GBM exhibit elevated Myc levels [9] . In addition, transgenic Myc expression in the astrocytic lineage of mice is sufficient to cause gliomas resembling the human disease [10] . Increased c-Myc activity downstream of p53 and Pten mutations is also causally associated with impaired neuronal differentiation and enhanced self-renewal capacity of GBM tumour-initiating cells [11] . Consistently, Myc knockdown in Pten −/− /p53 −/− double null neurospheres reduces their tumorigenic potential [11] . Others have proposed a central role for Myc also in the progression of gliomas driven by various different mutations [12] , [13] suggesting that Myc inhibition could be effective in multiple types of glioma. To assess the therapeutic potential of Myc inhibition in vivo we previously employed a dominant negative mutant of the Myc dimerization domain, termed Omomyc. Omomyc has an altered dimerization specificity, allowing it to sequester Myc away from its obligate partner Max and so inhibiting Myc-dependent transcriptional activation [14] , [15] . Making use of a TRE-Omomyc; CMVrtTA mouse model, in which Omomyc is widely expressed upon doxycycline administration [16] , we showed that systemic Myc inhibition triggers rapid regression of both KRas G12D -driven lung tumours [16] , [17] and T antigen-driven pancreatic β-cell insulinomas [18] in mice. Remarkably, such systemic Myc inhibition elicits only very mild and well-tolerated side effects in normal tissues [16] . Moreover, we observed no evolution of resistance to Myc inhibition in either tumour model, consistent with the unique and irreplaceable role Myc has as an integrator of proliferative transcriptional programs [17] . Here, we perform a comprehensive analysis of the therapeutic impact of systemic Myc inhibition in both progression and maintenance of glioma, comparing for the first time mouse and human experimental models, and investigate its actual mechanism of action. Myc inhibition increases survival of GFAP-V 12 Ha-Ras mice To determine the therapeutic impact of systemic Myc inhibition in both progression and maintenance of glioma, we combined our switchable TRE-Omomyc;CMVrtTA mouse with the well-characterized GFAP-V 12 Ha-Ras (ref. 19 ), a spontaneous mouse model of multifocal invasive astrocytoma in which the activated form of Ha-Ras is driven by the glial fibrillary acidic protein promoter (GFAP; Fig. 1a ). The molecular and pathological progression of disease in GFAP-V 12 Ha-Ras mice resembles that of diffuse astrocytomas in humans, exhibiting reproducible kinetics of tumour progression, from astroglial hyperplasia (starting from 1–3 weeks of age) through to low- and high-grade gliomas [20] . 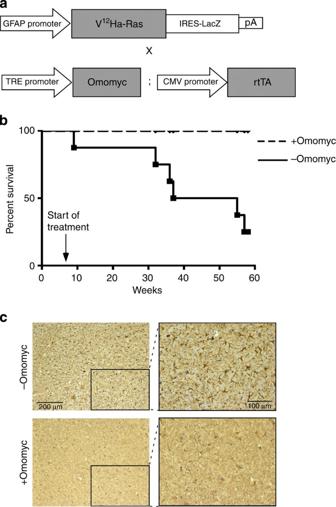Figure 1: Myc inhibition confers a survival advantage inGFAP-V12Ha-Rasmice. (a) To obtain a mouse model of spontaneous glioma in which Omomyc expression could be activated upon doxycycline treatment,TRE-Omomyc;CMVrtTAmice were crossed withGFAP-V12Ha-Rasmice, giving the triple transgenicTRE-Omomyc;CMVrtTA;GFAP-V12Ha-Ras.(b) Kaplan–Meier curve showing that Omomyc expression confers a significant survival advantage to V12Ha-Ras expressing mice. Eight-week-old mice, untreated or treated with Omomyc, were monitored for symptom-free survival up to 57 weeks of age.+Omomyc:TRE-Omomyc;CMVrtTA; GFAP-V12Ha-Rastriple transgenics plus doxycycline (n=8).−Omomyc: six vehicle-treatedTRE-Omomyc;CMVrtTA;GFAP-V12Ha-Rastriple transgenics and twoCMVrtTA;GFAP-V12Ha-Rastreated with doxycycline, to control for any doxycycline effect (n=8)P=0.014 by log-rank test. No effect of doxycycline was observed on tumour latency. (c) Representative pictures of GFAP immunostaining from the brains of mice included in the survival curve above. The panels on the right are higher magnification images of regions indicated by the black boxes. Control mice present dense GFAP-positive cells compared with Omomyc-treated mice. Figure 1: Myc inhibition confers a survival advantage in GFAP-V 12 Ha-Ras mice. ( a ) To obtain a mouse model of spontaneous glioma in which Omomyc expression could be activated upon doxycycline treatment, TRE-Omomyc;CMVrtTA mice were crossed with GFAP-V 12 Ha-Ras mice, giving the triple transgenic TRE-Omomyc;CMVrtTA;GFAP-V 12 Ha-Ras. ( b ) Kaplan–Meier curve showing that Omomyc expression confers a significant survival advantage to V 12 Ha-Ras expressing mice. Eight-week-old mice, untreated or treated with Omomyc, were monitored for symptom-free survival up to 57 weeks of age.+Omomyc: TRE-Omomyc;CMVrtTA; GFAP-V 12 Ha-Ras triple transgenics plus doxycycline ( n =8).−Omomyc: six vehicle-treated TRE-Omomyc;CMVrtTA;GFAP-V 12 Ha-Ras triple transgenics and two CMVrtTA;GFAP-V 12 Ha-Ras treated with doxycycline, to control for any doxycycline effect ( n =8) P =0.014 by log-rank test. No effect of doxycycline was observed on tumour latency. ( c ) Representative pictures of GFAP immunostaining from the brains of mice included in the survival curve above. The panels on the right are higher magnification images of regions indicated by the black boxes. Control mice present dense GFAP-positive cells compared with Omomyc-treated mice. Full size image Omomyc was induced in TRE-Omomyc;CMVrtTA ; GFAP-V 12 Ha-Ras mice from postnatal week 8 with doxycycline and the animals then monitored to determine symptom-free survival. Strikingly, at 57 weeks of age, all Omomyc-expressing mice (8/8) were asymptomatic with no evidence of disease progression ( Fig. 1b,c ). By contrast, at the same time point only 25% of the untreated control GFAP-V 12 Ha-Ras mice were still alive, the majority having been euthanized by this time point due to the appearance of progressive ataxia and neurological symptoms, associated with astrocytic hyperplasia and increased intracranial pressure ( Fig. 1c ). Of note, mice subjected continuously to Myc inhibition showed no sign of any distress or discomfort, confirming the previously reported well-tolerated and mild side effects elicited by Myc inhibition in normal tissue maintenance and homeostasis [16] . Myc inhibition limits growth of transformed neuroprogenitors To understand how Myc inhibition prevents glioma formation, we first investigated the cellular compartment previously identified in different glioma models as the putative cell of origin of the tumour: the neuroprogenitor (NPG) cells [21] , [22] . Recent reports demonstrate that glioma cells share features with neural stem and progenitor cells, including a high proliferation rate, and self-renewal and migration abilities [3] , [23] , [24] . As Myc has a demonstrated role in normal and neoplastic stem cell biology, we assessed the impact of Omomyc expression in primary NPG cells derived from our TRE-Omomyc;CMVrtTA;GFAP-V 12 Ha-Ras mice. Neural progenitor cells were isolated from the subventricular zones (SVZs) of either adult triple transgenic TRE-Omomyc;CMVrtTA;GFAP-V 12 Ha-Ras or control double transgenic TRE-Omomyc;CMVrtTA brains and grown as neurospheres in serum-free medium supplemented with growth factors (EGF and bFGF). As expected, the cells stayed strongly positive for GFAP expression ( Fig. 2a ). In these cultured NPGs, Omomyc mRNA expression was clearly detectable by 48 h of starting doxycycline treatment, whereas no Omomyc signal was detectable in untreated cells ( Supplementary Fig. 1 ). Of note, even though NPG cultures derived from the triple transgenic TRE-Omomyc; CMVrtTA;GFAP-V 12 Ha-Ras mouse expand significantly more than non-V 12 Ha-Ras-expressing TRE-Omomyc;CMVrtTA cells, Omomyc expression in Ras-transformed cells profoundly decreased total cell number at 3 days ( Fig. 2b ). At this same 3-day time point, the control cell culture had barely expanded and Omomyc expression had negligible effect on cell number ( Fig. 2c ). 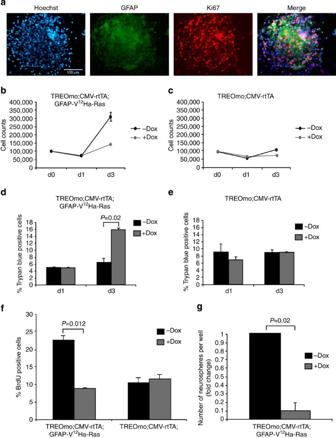Figure 2: Myc inhibition reduces proliferation and viability of V12Ha-Ras neuroprogenitors. (a) Neuroprogenitor cells freshly isolated from the subventricular zone (SVZ) of adult (3 months old) asymptomatic triple transgenicTRE-Omomyc;CMVrtTA;GFAP-V12Ha-Rascontrol mice were grown as neurospheres in culture in serum-free medium supplemented with growth factors (EGF and FGF). Immunostaining for GFAP (green) and Ki67 (red) are shown. Nuclei were counterstained with Hoechst (blue). (b,c) NPG growth curves. Neuroprogenitors were plated as single cells in 12-well plates and treated with doxycycline (+Dox) or untreated (–Dox) for 3 days. Triple transgenicTRE-Omomyc;CMVrtTA;GFAP-V12Ha-Rascells expressing Omomyc show a significant reduction in the total number of cells after 3 days of treatment, compared with the untreated cultures. (P-value=0.0168, calculated byt-test;b). Notably, 3 days of Omomyc expression in controlTRE-Omomyc;CMVrtTAdoes not affect significantly their growth rate (c). Data are shown as means±s.e. of triplicates (n=2). (d,e) Cell death was assessed by Trypan blue staining. Triple transgenicTRE-Omomyc;CMVrtTA;GFAP-V12Ha-RasNPGs have elevated numbers of dead cells after Omomyc expression for 3 days (d), whereas there is no difference in double transgenicTRE-Omomyc;CMVrtTANPGs (e). Data are shown as mean+s.e. of triplicates.P-values were calculated byt-test. (f) BrdU staining of triple transgenicTRE-Omomyc;CMVrtTA;GFAP-V12Ha-Rasand controlTRE-Omomyc;CMVrtTAcells treated with doxycycline for 3 days or untreated. Data represent the mean of triplicates+s.e. (n=3).P-values were calculated byt-test. (g) Omomyc expression impairs the self-renewal ability of triple transgenicTRE-Omomyc;CMVrtTA;GFAP-V12Ha-RasNPGs. Single neuroprogenitor cells were plated at a clonal density (500 per well) in a 12-well plate and treated or not with doxycycline. After 21 days, the number of spheres was evaluated. Data are shown as means+s.e. of triplicates (n=2).P-values were calculated byt-test. Figure 2: Myc inhibition reduces proliferation and viability of V 12 Ha-Ras neuroprogenitors. ( a ) Neuroprogenitor cells freshly isolated from the subventricular zone (SVZ) of adult (3 months old) asymptomatic triple transgenic TRE-Omomyc;CMVrtTA;GFAP-V 12 Ha-Ras control mice were grown as neurospheres in culture in serum-free medium supplemented with growth factors (EGF and FGF). Immunostaining for GFAP (green) and Ki67 (red) are shown. Nuclei were counterstained with Hoechst (blue). ( b , c ) NPG growth curves. Neuroprogenitors were plated as single cells in 12-well plates and treated with doxycycline (+Dox) or untreated (–Dox) for 3 days. Triple transgenic TRE-Omomyc;CMVrtTA;GFAP-V 12 Ha-Ras cells expressing Omomyc show a significant reduction in the total number of cells after 3 days of treatment, compared with the untreated cultures. ( P -value=0.0168, calculated by t -test; b ). Notably, 3 days of Omomyc expression in control TRE-Omomyc;CMVrtTA does not affect significantly their growth rate ( c ). Data are shown as means±s.e. of triplicates ( n =2). ( d , e ) Cell death was assessed by Trypan blue staining. Triple transgenic TRE-Omomyc;CMVrtTA;GFAP-V 12 Ha-Ras NPGs have elevated numbers of dead cells after Omomyc expression for 3 days ( d ), whereas there is no difference in double transgenic TRE-Omomyc;CMVrtTA NPGs ( e ). Data are shown as mean+s.e. of triplicates. P -values were calculated by t -test. ( f ) BrdU staining of triple transgenic TRE-Omomyc;CMVrtTA;GFAP-V 12 Ha-Ras and control TRE-Omomyc;CMVrtTA cells treated with doxycycline for 3 days or untreated. Data represent the mean of triplicates+s.e. ( n =3). P -values were calculated by t -test. ( g ) Omomyc expression impairs the self-renewal ability of triple transgenic TRE-Omomyc;CMVrtTA;GFAP-V 12 Ha-Ras NPGs. Single neuroprogenitor cells were plated at a clonal density (500 per well) in a 12-well plate and treated or not with doxycycline. After 21 days, the number of spheres was evaluated. Data are shown as means+s.e. of triplicates ( n =2). P -values were calculated by t -test. Full size image To determine the mechanism by which Omomyc expression blocks expansion of NPG cell cultures, we first examined cell death. Omomyc expression induced significant cell death in Ras-transformed NPGs but had no effect on the viability of control TRE-Omomyc;CMVrtTA cells ( Fig. 2d,e ). Omomyc also profoundly inhibited NPG proliferation: after 3 days of doxycycline treatment, we observed a significant reduction in the percentage of BrdU positive cells in TRE-Omomyc;CMVrtTA;GFAP-V 12 Ha-Ras NPGs, down to a rate similar to that observed in TRE-Omomyc;CMVrtTA controls, in which no difference was observed as a consequence of Omomyc expression ( Fig. 2f ). Hence, Omomyc exerts its effect on Ras-transformed cells both by reducing proliferation and enhancing cell death. Myc inhibition impairs NPG self-renewal capacity According to the cancer stem cell hypothesis, the refractoriness of gliomas to eradication by chemo- and radiotherapy is due to a subpopulation of cells within the tumour that has stem cell features, including a high proliferation rate and self-renewal capacity. To investigate whether Myc inhibition impairs these characteristics, we employed a neurosphere self-renewal assay, measuring the number of cells able to reform a secondary neurosphere from a single cell. In this assay, NPGs are seeded at clonal density (500 single cells per well), then cultured with or without doxycycline for 21 days, at which point the number of spheres in each well is determined. Notably, Omomyc expression impairs the self-renewal ability of both the Ras-transformed and the control cells ( Fig. 2g and Supplementary Fig. 1b ), consistent with the crucial role ascribed to Myc proteins in promoting and maintaining self-renewal and stemness of both neoplastic and normal progenitor cells [25] , [26] . Myc inhibition reverses the symptoms of GFAP-V 12 Ha-Ras mice To test the therapeutic utility of Myc inhibition in advanced gliomas, we evaluated the impact of Omomyc expression in TRE-Omomyc;CMVrtTA;GFAP-V 12 Ha-Ras mice presenting already clear neurological symptoms. Due to the variable tumour latency of our colony (see Fig. 1b , untreated–Omomyc animals), such symptoms appeared stochastically: the animals were initially hyperactive and often aggressive, but eventually became almost catatonic and unresponsive to external stimuli. At this point, they were treated with Omomyc. After 7 days of Myc inhibition, the therapeutic effect was dramatic. As documented by the movie ( Supplementary Movie 1 ), mice were typically lethargic at the commencement of treatment, failed to groom and lacked appetite. After 7 days of Myc inhibition however, treated mice were active, responded again to external stimuli and were able to move, eat, drink and groom ( Supplementary Movie 2 ). Histological analysis of treated versus untreated samples clearly showed that untreated symptomatic mice exhibited regions with high density, GFAP-positive, pleomorphic and infiltrative astrocytes, typical histopathological features of human malignant astrocytomas ( Fig. 3 , middle versus upper panels). By contrast, the improved health of treated animals was associated with markedly reduced astrocytic (GFAP positive) cell density ( Fig. 3 , lower panels). Further immunohistochemical analysis of the residual GFAP-positive regions in Myc-inhibited symptomatic mice revealed a significant decrease in the number of proliferating cells compared with untreated mice (3.63% versus 7.83% positivity for the proliferation marker Ki67; Fig. 4a,b ). In addition, we noted a small but significant increase in the number of apoptotic (TUNEL-positive) cells in Omomyc-expressing mouse brains when compared with Omomyc-negative controls (1.74% versus 0.48%; Fig. 4a,c ), indicating that cell death contributes—at least to some degree—to the reduced cellular density observed upon Myc inhibition. A notable reduction in total cell number after Omomyc expression was confirmed by determining the number of nuclei present in five whole macroscopic fields (see total number of nuclei in treated versus untreated animals in Fig. 4b,c ). 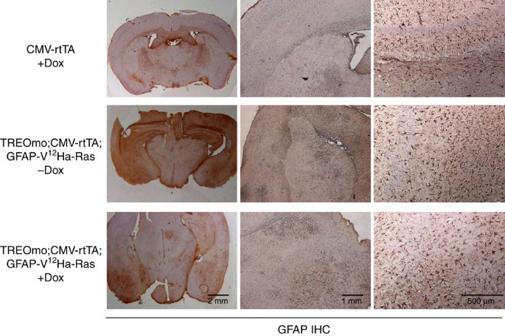Figure 3: Histological analysis of symptomatic mice. Representative GFAP immunostaining of normalCMVrtTAand triple transgenicTRE-Omomyc;CMVrtTA;GFAP-V12Ha-Rasbrains. Left panels show that astrocytic density is reduced in Omomyc-expressing mice. Center panels focus on residual GFAP-positive regions. Right panels show higher magnification of astrocytes and active microglia. Figure 3: Histological analysis of symptomatic mice. Representative GFAP immunostaining of normal CMVrtTA and triple transgenic TRE-Omomyc;CMVrtTA;GFAP-V 12 Ha-Ras brains. Left panels show that astrocytic density is reduced in Omomyc-expressing mice. Center panels focus on residual GFAP-positive regions. Right panels show higher magnification of astrocytes and active microglia. 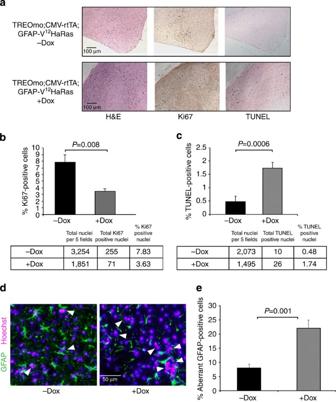Figure 4: Effects of Myc inhibition in the brain ofGFAP-V12Ha-Rassymptomatic mice. (a) Symptomatic triple transgenicTRE-Omomyc;CMVrtTA;GFAP-V12Ha-Rasmice were treated with doxycycline for 7 days (n=2) or untreated (n=3). Histological analysis (left panels) shows a reduction in Ki67 positive (proliferating) cells and an increase in dying TUNEL-positive cells in Omomyc-expressing mice. (b) Quantification of the Ki67 positivity from the histological analysis ina. The percentage of proliferating cells is shown in the graph, and the total number of cells counted in five fields is also indicated in the table. (c) Quantification of the TUNEL positivity from the histological analysis described above. The percentage of TUNEL-positive cells is shown in the graph, and the total number of cells counted in five fields is also indicated in the table. (d) Omomyc treatment causes the appearance of multinucleated cells. Symptomatic triple transgenicTRE-Omomyc;CMVrtTA;GFAP-V12Ha-Rasmice were treated with doxycycline for 7 days. Histological analysis was performed on isolated brains to look for GFAP-positive astrocytes in tumour regions (green dye). Nuclei were counterstained with Hoechst (coloured pink here after merging with the GFAP images to facilitate visualization of the nuclei). (e) Quantification of the number of multinucleated GFAP-positive nuclei after Omomyc treatment (n=2) for 7 days compared with untreated mice (n=2). The average of two mice is shown+s.e. For each mouse, a minimum of 10 microscopic fields and 300 cells were scored. Data are shown as means+s.e.P-value was calculated by Student’st-test. Full size image Figure 4: Effects of Myc inhibition in the brain of GFAP-V 12 Ha-Ras symptomatic mice. ( a ) Symptomatic triple transgenic TRE-Omomyc;CMVrtTA;GFAP-V 12 Ha-Ras mice were treated with doxycycline for 7 days ( n =2) or untreated ( n =3). Histological analysis (left panels) shows a reduction in Ki67 positive (proliferating) cells and an increase in dying TUNEL-positive cells in Omomyc-expressing mice. ( b ) Quantification of the Ki67 positivity from the histological analysis in a . The percentage of proliferating cells is shown in the graph, and the total number of cells counted in five fields is also indicated in the table. ( c ) Quantification of the TUNEL positivity from the histological analysis described above. The percentage of TUNEL-positive cells is shown in the graph, and the total number of cells counted in five fields is also indicated in the table. ( d ) Omomyc treatment causes the appearance of multinucleated cells. Symptomatic triple transgenic TRE-Omomyc;CMVrtTA;GFAP-V 12 Ha-Ras mice were treated with doxycycline for 7 days. Histological analysis was performed on isolated brains to look for GFAP-positive astrocytes in tumour regions (green dye). Nuclei were counterstained with Hoechst (coloured pink here after merging with the GFAP images to facilitate visualization of the nuclei). ( e ) Quantification of the number of multinucleated GFAP-positive nuclei after Omomyc treatment ( n =2) for 7 days compared with untreated mice ( n =2). The average of two mice is shown+s.e. For each mouse, a minimum of 10 microscopic fields and 300 cells were scored. Data are shown as means+s.e. P -value was calculated by Student’s t -test. Full size image Intriguingly, we observed that in the GFAP-positive regions remaining after Omomyc treatment, there was a significant increase in multinucleated GFAP-positive cells compared with untreated animals, suggestive of an effect of Myc inhibition on ploidy and mitosis of astrocytoma cells ( Fig. 4d,e ). Myc inhibition triggers mitotic crisis in human GBM cells To ascertain whether the antitumorigenic effect of Myc inhibition in the mouse model might translate into an analogous therapeutic impact in a human system, we investigated the effect of Omomyc expression in cell lines derived from human grade IV gliomas. U87MG cells [27] were infected with retroviruses directing the expression of either GFP (control) or a GFP-Omomyc fusion protein. Consistent with our in vivo results in the GFAP-V 12 Ha-Ras mouse model, the total U87MG cell number was reduced on Omomyc induction, whereas GFP expression alone had no such effect ( Fig. 5a ). In addition, we observed a significant increase in cell death in U87MG cells expressing Omomyc, compared with control cells ( Fig. 5b ). Using a doxycycline-switchable lentiviral vector to drive expression of Omomyc, we also observed an increase in the proportion of flattened, senescent-like cells that stained positively for β-galactosidase ( Fig. 5c ). Broadly similar observations were made in Omomyc-expressing U373MG cells, which notably are mutant for p53 ( Supplementary Fig. 2 ), although the cell flattening seen in U87MG cultures after Omomyc expression was not recapitulated ( Supplementary Fig. 2c ). 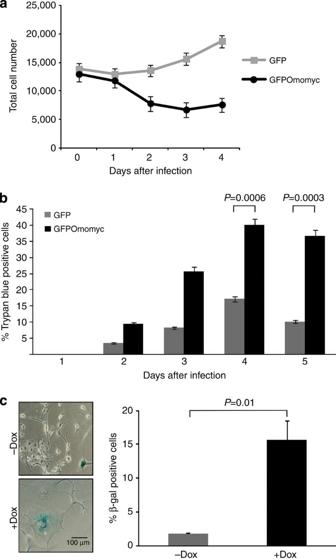Figure 5: Omomyc causes growth arrest and increases cell death in U87MG cells. (a) Growth curves of U87MG infected with GFP control or GFP-Omomyc-expressing retroviruses. Total cell number was quantified at the indicated time points. Data are shown as the mean±s.e. of triplicates from a single experiment representative of three repeats.P-value at 3 days <0.05;P-value at 4 days <0.01, using a two-tailedt-test. (b) Cell death was assessed by Trypan blue staining. The number of dead cells was quantified at the indicated time points. Data are shown as mean±s.e. of triplicates.P-values were calculated byt-test. (c) U87MG cells were infected with a doxycycline-switchable lentiviral vector expressing Omomyc. Doxycycline treatment increases the number of β-galactosidase positive, senescent-like cells (left panels: typical β-galactosidase phase contrast images, right panel: quantification). The average of three experiments+s.d. is shown.P-values were calculated by a Student’st-test. Figure 5: Omomyc causes growth arrest and increases cell death in U87MG cells. ( a ) Growth curves of U87MG infected with GFP control or GFP-Omomyc-expressing retroviruses. Total cell number was quantified at the indicated time points. Data are shown as the mean±s.e. of triplicates from a single experiment representative of three repeats. P -value at 3 days <0.05; P -value at 4 days <0.01, using a two-tailed t -test. ( b ) Cell death was assessed by Trypan blue staining. The number of dead cells was quantified at the indicated time points. Data are shown as mean±s.e. of triplicates. P -values were calculated by t -test. ( c ) U87MG cells were infected with a doxycycline-switchable lentiviral vector expressing Omomyc. Doxycycline treatment increases the number of β-galactosidase positive, senescent-like cells (left panels: typical β-galactosidase phase contrast images, right panel: quantification). The average of three experiments+s.d. is shown. P -values were calculated by a Student’s t -test. Full size image Cytological examination of fixed Omomyc-expressing U87MG cells stained for tubulin and DNA showed that Omomyc expression causes a reduction in the mitotic index (0.96% versus 1.86% in control cells), but does not affect mitotic progression (the prophase+metaphase/anaphase+telophase ratio was 0.317 in Omomyc-expressing cells and 0.326 in GFP-expressing cells). A fraction of the dividing cells in Omomyc-expressing cultures (14.7%) displayed mitotic defects including multipolar spindles, aberrant chromosome segregation, chromatin bridges in ana-telophase and an irregular central spindle/midbody ( Fig. 6a (control cells) versus Fig. 6b (Omomyc-expressing cells)). The final outcome of these defective mitoses was the formation of multinucleated and micronuclei-containing cells (13.6% after 72 h Omomyc expression; Fig. 6c,d , and Supplementary Fig. 3a ). Similar results were obtained in U373MG cells with a doxycycline-switchable RFP-Omomyc-expressing vector ( Supplementary Fig. 3b and c ), where time-lapse imaging over the course of 72 h revealed that multinucleated cells enter mitosis but are unable to complete the mitotic process and may eventually die ( Supplementary Movie 3 ). 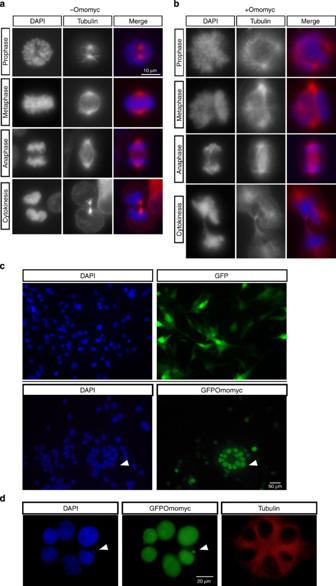Figure 6: Myc inhibition triggers micro- and multinucleation and mitotic abnormalities in U87MG cells. (a) Normal mitosis phases in control U87MG cells. Tubulin staining (second column and in red in the merged image) shows proper centrosome maturation and spindle assembly, whereas DAPI staining (first column and in blue in the merged image) highlights correct chromosome alignment and subsequent segregation. (b) Mitotic defects in Omomyc-expressing cells. The same tubulin and DAPI staining as above show that Omomyc induces defects in all mitotic phases, ranging from abnormal multipolar spindles (prophase and metaphase panels), to chromosome misalignments, segregation errors and lagging chromosomes (anaphase and cytokinesis panels), and finally absence of midbody and failed cytokinesis (bottom panel). Mitotic abnormalities involve 14.7% of mitotic figures in Omomyc-expressing cells. (c) GFP (green) immunofluorescence and DAPI nuclear counterstain (blue) show that after 24 h of GFP-Omomyc expression, U87MG cells become multinucleated (bottom panels) whereas that is observed much less frequently in control U87MG (top panel) that express GFP alone. (d) A representative image of a multinucleated Omomyc-expressing cell: α-tubulin staining (in red) shows that all nuclei belong to the same cell. The arrowhead indicates a typical micronucleus. Figure 6: Myc inhibition triggers micro- and multinucleation and mitotic abnormalities in U87MG cells. ( a ) Normal mitosis phases in control U87MG cells. Tubulin staining (second column and in red in the merged image) shows proper centrosome maturation and spindle assembly, whereas DAPI staining (first column and in blue in the merged image) highlights correct chromosome alignment and subsequent segregation. ( b ) Mitotic defects in Omomyc-expressing cells. The same tubulin and DAPI staining as above show that Omomyc induces defects in all mitotic phases, ranging from abnormal multipolar spindles (prophase and metaphase panels), to chromosome misalignments, segregation errors and lagging chromosomes (anaphase and cytokinesis panels), and finally absence of midbody and failed cytokinesis (bottom panel). Mitotic abnormalities involve 14.7% of mitotic figures in Omomyc-expressing cells. ( c ) GFP (green) immunofluorescence and DAPI nuclear counterstain (blue) show that after 24 h of GFP-Omomyc expression, U87MG cells become multinucleated (bottom panels) whereas that is observed much less frequently in control U87MG (top panel) that express GFP alone. ( d ) A representative image of a multinucleated Omomyc-expressing cell: α-tubulin staining (in red) shows that all nuclei belong to the same cell. The arrowhead indicates a typical micronucleus. Full size image Myc inhibition alters SAE1 expression and PTP1B phosphorylation Loss of SUMO activating enzyme (SAE) expression was recently found to exhibit synthetic lethality together with Myc overexpression [28] . One intriguing phenotypic outcome of SAE knockdown in Myc overexpressing tumour cells was the appearance of mitotic abnormalities and induction of mitotic catastrophe [28] . Interestingly, SAE1 is a direct target of Myc [29] . To verify whether SAE1 could be altered in response to Omomyc expression, we performed western blot analysis on GBM cell lines. We observed a clear reduction of SAE1 expression in U87MG ( Fig. 7a ). Hence, reduced SAE activity could be responsible for the aberrant nuclei and mitotic catastrophe observed in this cell line. 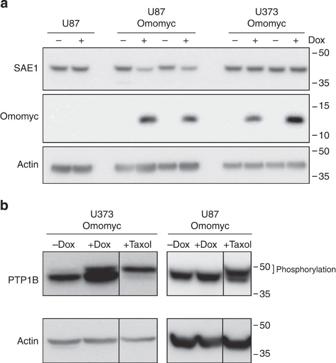Figure 7: Omomyc causes alterations in proteins linked to mitotic cell death. (a) Western blot analysis of samples from GBM cells shows that Omomyc causes a decrease in SAE1 expression in U87MG but not U373MG cells. GBM cells with a lentiviral Omomyc expression cassette were treated with doxycycline for 6 days to induce Omomyc expression. Two independent sets of samples are shown for each of the GBM cell lines. (b) Western blot analysis of GBM samples shows that Omomyc expression triggers an increase in PTP1B phosphorylation in U373MG cells. GBM cells with a lentiviral Omomyc expression cassette were treated with doxycycline for 6 days to induce Omomyc expression. A Taxol control was used to indicate the typical phosphorylation-induced mobility shift of PTP1B during mitotic catastrophe. Taxol-treated control samples are nonadjacent bands from the same western blot. Figure 7: Omomyc causes alterations in proteins linked to mitotic cell death. ( a ) Western blot analysis of samples from GBM cells shows that Omomyc causes a decrease in SAE1 expression in U87MG but not U373MG cells. GBM cells with a lentiviral Omomyc expression cassette were treated with doxycycline for 6 days to induce Omomyc expression. Two independent sets of samples are shown for each of the GBM cell lines. ( b ) Western blot analysis of GBM samples shows that Omomyc expression triggers an increase in PTP1B phosphorylation in U373MG cells. GBM cells with a lentiviral Omomyc expression cassette were treated with doxycycline for 6 days to induce Omomyc expression. A Taxol control was used to indicate the typical phosphorylation-induced mobility shift of PTP1B during mitotic catastrophe. Taxol-treated control samples are nonadjacent bands from the same western blot. Full size image On the other hand, in U373MG cells we observed no downregulation of SAE1 ( Fig. 7a ). Instead, phosphorylation of protein tyrosine phosphatase 1B (PTP1B)—a modification associated with and required for cell death during mitotic catastrophe [30] —was observed in response to Myc inhibition ( Fig. 7b ), to a degree similar to that caused by Taxol, a well-characterized microtubule stabilizer and mitosis inhibitor previously shown to cause PTP1B phosphorylation [30] . These results offer at least two new potential mechanisms for Omomyc-induced cell death in GBM and hint at yet another aspect of proliferative biology in which Myc is involved. Myc inhibition limits growth of patient-derived tumours To determine whether the antitumorigenic capacity of Myc inhibition extends to primary human tumour samples and, consequently, might be clinically applicable in human glioma, we used a lentiviral vector to drive doxycycline-dependent Omomyc expression in patient-derived GBM neurosphere cultures derived from a surgically resected human GBM ( Supplementary Fig. 4a ). In culture, Myc inhibition for 2 weeks reduced the overall number of neurospheres ( Fig. 8a ) and inhibited self-renewal of spheres after their dissociation ( Fig. 8b ). No effect of doxycycline treatment was observed in neurospheres lacking the Omomyc lentiviral vector ( Supplementary Fig. 4b ). 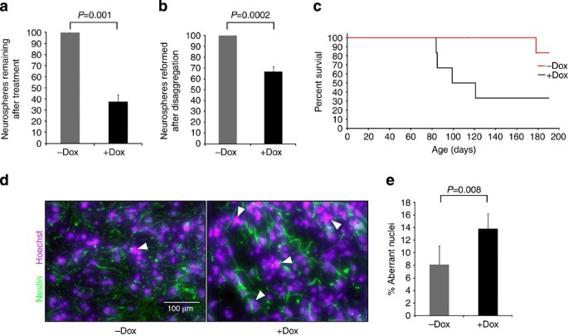Figure 8: Myc inhibition decreases the growth of patient-derived neurospheresin vitroand increases the survival of a xenograft mouse model. (a) Patient-derived neurosphere cultures derived from a resected human glioblastoma were infected with a lentiviral vector harbouring a doxycycline-regulatable Omomyc expression cassette. Myc inhibition by Omomyc decreases the number of spheres after 2 weeks of doxycycline treatment in culture. The mean+s.e.m. is shown (n=6).P-values were calculated by a Student’st-test. (b) Omomyc expression in disaggregated neurospheres decreases their self-renewal ability. Neurospheres were dissociated into a single-cell suspension and 500 cells per well were added to a 96-well plate. The number of spheres was counted after 2–4 weeks in the presence or absence of doxycycline. The mean+s.e.m. is shown (n=5).P-values were calculated by a Student’st-test. (c) A Kaplan–Meier survival curve of mice inoculated with patient-derived neurospheres and treated with doxycycline to trigger Omomyc expression (n=6), or with sucrose as the control (n=6).P=0.04 by log-rank test. (d) Omomyc expression increases the number of aberrant nuclei in nestin-positive cells. At the time of euthanasia, brains of the orthotopically injected mice described in 8cwere fixed, and sections stained for nestin. Typical images are shown (green: nestin, pink: Hoechst). (e) Quantification of the experiment described in 8d. Five sections taken from different parts of each brain were used to score the number of aberrant nestin-positive nuclei (indicated by arrowheads). Untreated micen=4, treated with doxycyclinen=5.P-values were calculated by a Student’st-test. Figure 8: Myc inhibition decreases the growth of patient-derived neurospheres in vitro and increases the survival of a xenograft mouse model. ( a ) Patient-derived neurosphere cultures derived from a resected human glioblastoma were infected with a lentiviral vector harbouring a doxycycline-regulatable Omomyc expression cassette. Myc inhibition by Omomyc decreases the number of spheres after 2 weeks of doxycycline treatment in culture. The mean+s.e.m. is shown ( n =6). P -values were calculated by a Student’s t -test. ( b ) Omomyc expression in disaggregated neurospheres decreases their self-renewal ability. Neurospheres were dissociated into a single-cell suspension and 500 cells per well were added to a 96-well plate. The number of spheres was counted after 2–4 weeks in the presence or absence of doxycycline. The mean+s.e.m. is shown ( n =5). P -values were calculated by a Student’s t -test. ( c ) A Kaplan–Meier survival curve of mice inoculated with patient-derived neurospheres and treated with doxycycline to trigger Omomyc expression ( n =6), or with sucrose as the control ( n =6). P =0.04 by log-rank test. ( d ) Omomyc expression increases the number of aberrant nuclei in nestin-positive cells. At the time of euthanasia, brains of the orthotopically injected mice described in 8 c were fixed, and sections stained for nestin. Typical images are shown (green: nestin, pink: Hoechst). ( e ) Quantification of the experiment described in 8 d . Five sections taken from different parts of each brain were used to score the number of aberrant nestin-positive nuclei (indicated by arrowheads). Untreated mice n =4, treated with doxycycline n =5. P -values were calculated by a Student’s t -test. Full size image To investigate whether this potentially therapeutic effect might translate into an objective therapeutic impact, disaggregated neurospheres were orthotopically inoculated into the brains of NOD/SCID mice. Animals transplanted with neurospheres harbouring the Omomyc expression cassette were treated continuously with either doxycycline from 3 weeks after transplant (so that Omomyc was expressed throughout tumour development) or with sucrose in control mice. As expected, Myc inhibition significantly potentiated overall survival ( Fig. 8c ). Importantly, once again, we observed the appearance of aberrant nuclei in nestin-positive cells after Omomyc treatment ( Fig. 8d,e ). We previously demonstrated in preclinical mouse models that systemic Myc inhibition is a promising strategy for eradicating lung cancer [16] , [17] and insulinoma [18] , inducing profound regression of tumours, eliciting only very mild side effects in normal tissues and circumventing the problems with resistance encountered in other targeted therapies. However, whether or not these conclusions were applicable to other types of cancer and to human cancers remained to be established. Here, we extend our previous studies by showing that Myc inhibition has a similar effective therapeutic potential for treating glioma, a disease with an especially dismal prognosis and in urgent need of new therapies. To do this, we made use of several experimental models, encompassing both mouse and human systems, including a Ras-driven mouse model of astrocytoma and NPG cells derived from it, human GBM cell lines and, importantly, a patient-derived neurosphere xenograft model. All these studies, both in vitro and in vivo , indicate that Myc inhibition suppresses glioma formation, inhibits glioma cell proliferation and survival and triggers regression of established disease. Unexpectedly, we also noted that Myc inhibition elicits profound aberrations in glioma cell mitosis, with the appearance of multinucleated cells, micronucleation and also multipolar and disorganised spindles. Time-lapse microscopy confirmed that such aberrant mitotic cells are unable to complete cell division and many subsequently die. Although the suppression of Myc might be expected to induce replicative arrest—given its intimate role in coordinating cell proliferation—the mechanisms underlying glioma cell mitotic dysfunction and death are particularly intriguing. Interestingly, SUMO pathway components have been shown to be required for cell division and implicated in the control of mitotic chromosome structure, cell cycle progression, kinetochore function and cytokinesis [31] . Here we show that SAE1, a direct target of Myc [29] , is downregulated in response to Omomyc expression in U87MG cells ( Fig. 7a ), suggesting that a reduction in SAE activity is responsible for the aberrant nuclei and mitotic catastrophe observed in this cell line. In contrast, U373MG cells display no such downregulation of SAE1 levels but Myc inhibition is instead associated with the phosphorylation of PTP1B, a modification described to trigger cell death during mitotic catastrophe [30] . The phosphatase PTP1B has been recently shown to exert antitumour effects in GBM [32] , however, it displays tumour-promoting effects in other cell types; opposing functions may be controlled by posttranslational modifications and substrate specificity. For example, PTP1B is negatively regulated by sumoylation upon entry into mitosis [33] , whereas its phosphorylation by Cdk1 and Plk1 during mitotic arrest promotes its activation and tumour suppressing activity [30] . Details of how these opposing modifications interact to determine cell fate remain unknown. In this study we provide evidence to support the hypothesis that Myc inhibition blocks protein sumoylation (via decreased SAE1 expression) leading to defective mitosis, and ultimately the induction of mitotic catastrophe. Failure to satisfy the spindle assembly checkpoint (SAC) results in protracted M-phase arrest and sustained activation of mitotic kinases, leading to death during mitosis. In addition, enhanced PTP1B activity as a result of Omomyc-dependent loss of PTP1B sumoylation and consequent gain in its phosphorylation may also directly contribute to mitotic cell death. Our results demonstrate that Myc holds a central role in proficient mitotic programs, the precise molecular mechanism of which could vary in different cell types depending on the status of other cell cycle or genome integrity regulators, such as p53. It isnot surprising that the pleiotropic nature of Myc is reflected in the degeneracy of its effectors, some of which control programs necessary for efficient cell division. Whether or not the effects of Myc inhibition on mitotic aberrations are peculiar to GBM cells or also hold in other types of cancer remains to be established. The mode of action of a Myc inhibitor—in our case Omomyc—could vary with the context-specific role of Myc, whose function ramifies throughout all aspects of tumorigenesis both at the intracellular and the extracellular levels. Our data demonstrate that systemic Myc inhibition appears to be a very promising strategy for treating glioma, seemingly irrespective of its driving oncogenic lesions. While direct inhibition of Myc is currently not a pharmacological option, it may in the future prove possible to inhibit Myc function, either directly as recently shown using peptides derived from Myc itself [12] or indirectly, as demonstrated for bromodomain inhibitors [34] . Study design All the animal studies were performed in accordance with ARRIVE guidelines and following the three R’s rule of Replacement, Reduction and Refinement principles. Mice were housed and treated in accordance with protocols approved by the Institutional Animal Care and Use Committee at the UCSF (University of California, San Francisco) and by the CEEA (Ethical Committee for the Use of Experimental Animals) at the VHIO (Vall d’Hebron Institute of Oncology), Barcelona. The anonymized human sample employed was part of the tissue biological material stored in the tumour bank (TB) at the Hospital Vall d’Hebron. The sample had been previously collected with a signed patient consent form and its use had been approved by the Ethics Committee of the Hospital. The sample was a random one among the GBM patient samples available. Generation and maintenance of mice TRE -Omomyc;CMVrtTA mice were previously described [16] . GFAP-V 12 Ha-Ras ( Tg(GFAP-Hras1)1Agu ) mice were generated and kindly provided by Dr Abhijit Guha (Toronto Hospital Western Division-UHN) and Dr David H. Gutmann (WUSM) laboratories. The resulting triple transgenic TRE-Omomyc;CMVrtTA;GFAP-V 12 Ha-Ras mice were of a mixed CD1;FVB/N;C57BL/6 background. Doxycycline was dissolved in drinking water (2 mg ml −1 with 5% sucrose) and administered to the animals. Control animals received 5% sucrose. Tissue preparation and histology Mouse brains were removed and either frozen in OCT or fixed overnight in Zinc-buffered formalin and processed for paraffin embedding. For histological analysis, tissue sections (5 μm) were stained with haematoxylin and eosin. Immunohistochemistry For immunohistochemical analysis, tissue sections were de-paraffinized, rehydrated and subjected to high temperature antigen retrieval in 10 mM citrate buffer (pH 6.0). The following primary antibodies were used: rabbit monoclonal anti-Ki67 (clone SP6, Lab Vision, 1:100) rabbit polyclonal anti-GFAP (Novus Biologicals, 1:100), anti-nestin (Millipore, 1:100). These primary antibodies were applied for 2 h in blocking buffer (2.5% BSA, 5% goat serum, 0.3% Triton X-100 in PBS), followed by species-appropriate secondary Alexa Fluor 488 dye conjugated antibodies (Amersham) or Vectastain ABC kit and DAB reagents (Vector Laboratories). Fluorescence antibody-labeled slides were mounted in DAKO fluorescent mounting medium containing 1 μg ml −1 Hoechst counterstain. HRP-conjugated secondary antibodies were visualized by DAB staining (Vector Laboratories). Apoptotic cells were detected with ApopTag Detection kit (Chemicon International). Images were obtained with an Axiovert S100 TV inverted fluorescence microscope (Zeiss) and Open Lab 3.5.1 software, or with an Axiovert 100 inverted microscope (Zeiss) equipped with a Hamamatsu Orca digital camera. NPG isolation and culture NPGs were isolated from the SVZ of adult mice. Brains were dissected and washed in Hank’s buffer (Gibco). Tissue samples were minced, digested for 40 min with 0.05% trypsin, triturated and passed through a 45 μm cell strainer (BD Biosciences) to obtain a single-cell suspension. Cells were seeded in serum-free neurobasal medium (Gibco) supplemented with 20 ng ml −1 of Human bFGF (Gibco), 20 ng ml −1 EGF (Sigma), Heparin (Sigma), B27 (Gibco), pen/strep and glutamine. Cells were grown at 37 °C in 5% CO 2 . NPG cell growth, Trypan blue exclusion assay and BrdU staining A total of 10 5 cells were seeded in triplicate in 12-well plates. They were then counted daily using a Neubauer hemocytometer for 3 days, and cell death was estimated by Trypan blue dye exclusion assay. On the third day, cells were incubated for 5 h with the BrdU substrate (Roche), collected and fixed overnight in 70% ethanol. Staining with the BrdU antibody (BD Biosciences) was performed following the manufacturer’s instructions. Cells were then counterstained with propidium iodide and analysed with a FacsCanto flow cytometer (BD Biosciences). Analysis was performed using FlowJo software. NPG immunofluorescence NPGs were centrifuged with CytoSpin (Eppendorf) to cause them to adhere onto slides and fixed in 4% paraformaldehyde. Fixed cells were blocked with 5% BSA–0.1% Triton and then incubated with rabbit monoclonal anti-Ki67 (clone SP6, Lab Vision, 1:100) and rabbit polyclonal anti-GFAP (Novus Biologicals, 1:500) overnight and counterstained with Hoechst. Images were collected with an Axiovert S100 TV inverted fluorescence microscope (Zeiss) and Open Lab 3.5.1 software. NPG self-renewal assay To evaluate the self-renewal capacity of NPGs, a clonal colony-forming assay was used to measure the proportion of cells that were able to make new neurospheres. Single-cell dissociated NPGs were seeded in triplicate into 24- or 96-well plates with 500 cells per well, and the number of newly formed neurospheres was counted after 3–4 weeks. β-galactosidase staining β-galactosidase staining was performed as described in the protocol (Cell Signaling). GBM cells were incubated for 2 days in the presence of X-gal to visualize the positive blue cells. RNA and protein analysis Cells grown and treated or not with doxycycline for 3 days were either used for RNA extraction with a RNAeasy kit (Qiagen) according to manufacturer’s instructions, or lysed in RIPA buffer with proteases and phosphatases inhibitors (Roche). RNA was retro-transcribed with the iScript cDNA Synthesis Kit (Bio-Rad) and quantitative PCR with reverse transcription was performed using the following Taqman probe for Omomyc: 5′-/56- FAM/ATTTCAGAAATGAGCTTTTGCGTCTC /36-TAMSp/-3′. Protein extracts were run on 10% or 12% precast gels (Life Technologies), transferred to PVDF membranes (Millipore) and incubated with antibodies against SAE1 (Novus Biologicals, 1:1,000), PTP1B (BD Biosciences, 1:2,000), FLAG (Sigma, 1:4,000) or actin (Sigma, 1:200,000). Complete western blot images are included as Supplementary Fig. 5 . U87MG and U373MG culture Human GBM U87MG and U373MG cell lines were maintained in Dulbecco’s Modified Eagle’s medium supplemented with 10% fetal bovine serum, glutamine (2 mM), penicillin (50 units ml −1 ), and streptomycin (50 g ml −1 ) at 37 °C in 5% CO 2 . For growth curves and cell viability assays, 10 4 cells were seeded in triplicate in 24-well plates. Cells were counted daily using a Neubauer hemocytometer for 5 days, while cell death was quantified by Trypan blue dye exclusion assay. For the quantification of multinucleated cells, cells were seeded and fixed with 4% paraformaldehyde on coverslips 48, 72 and 120 h after the infection with retroviruses producing either GFP or the fusion protein GFP-Omomyc. Cells were then mounted on microscope slides with 4′,6-diamidino-2-phenylindole (DAPI)-containing Vectashield mounting solution. Images of around 2,000 cells were acquired using a fluorescence microscope (Zeiss) with a × 20 objective. The number of total and GFP+ cells with a number of nuclei >3 were counted. For mitosis analysis, cells were seeded on coverslips in a six-well plate and fixed 72 h after the infection with retroviruses producing either GFP or the fusion protein GFP-Omomyc. Cells were then permeabilized in PBS containing 0.2% Triton X-100 and blocked in 5% BSA. α-Tubulin was detected using a mouse monoclonal primary antibody (Sigma, T9026, 1:100) and a Cy3 secondary antibody (Jackson ImmunoResearch, 1:10). After immunostaining, cells were mounted on microscope slides with DAPI-containing Vectashield mounting solution (Vector Laboratories). For both Omomyc-expressing and control cells, images of 48 different mitoses were acquired using a fluorescence microscope (Zeiss) with a × 63 objective. Viral vectors and infections Omomyc DNA was cloned into the pEGFP retroviral vector (Clontech). A total of 2.5 × 10 6 293T cells were seeded on 60-mm plates and co-transfected with packaging plasmids Plp1, Plp2, PlpV/SVG (Invitrogen) and pEGFP or pEGFP-Omomyc retroviral constructs using CaPO 4 method. Supernatant was collected twice during the 2 days following transfection. The day before transfection, 1.5 × 10 6 U87MG cells were seeded on 35-mm plates. Cells were then infected with 293T cells-derived supernatant containing retroviruses and polybrene (4 μg ml −1 ). Omomyc was cloned into the pTRIPZ lentiviral vector (Open Biosystems, Thermo Scientific) and the shRNA sequences removed. For infections, 293T cells were seeded at 70% confluence and the following morning 25 μM chloroquinone added. Two hours later, 293 cells were transfected with pTRIPZ-Omomyc plus the lentiviral vectors pMD2G and psPAX2 by the CaPO 4 method. The medium was changed the following day and sodium butyrate added at 5 mM. Viral supernatants were harvested on the subsequent 2 days, filtered and added to target cells with polybrene (0.8 μg ml −1 ). Patient-derived neurosphere culture and orthotopic inoculation Neurospheres were isolated, cultured and inoculated as described previously [35] . Briefly, tumour cells from disaggregated patient-derived neurospheres were stereotactically inoculated into the corpus striatum of the right brain hemisphere (1 mm anterior and 1.8 mm lateral to the bregma; 2.5 mm intraparenchymal) of 9-week-old NOD-SCID mice (Charles River Laboratories). Three weeks after transplantation, the animals received doxycycline dissolved in drinking water (2 mg ml −1 with 5% sucrose). Control animals received only sucrose. Mice were euthanized when they presented with neurological symptoms or a significant loss of weight. Statistical analysis Data are shown in bar graphs as means+standard deviation (s.d. ), or as standard error (s.e.) if indicated. P -values were calculated using Student’s t -test to compare groups, or log-rank test for Kaplan–Meier curves. How to cite this article: Annibali, D. et al . Myc inhibition is effective against glioma and reveals a role for Myc in proficient mitosis. Nat. Commun. 5:4632 doi: 10.1038/ncomms5632 (2014).